Direct visualization of cell division using high-resolution imaging of M-phase of the cell cycle Current approaches to monitor and quantify cell division in live cells, and reliably distinguish between acytokinesis and endoreduplication, are limited and complicate determination of stem cell pool identities. Here we overcome these limitations by generating an in vivo reporter system using the scaffolding protein anillin fused to enhanced green fluorescent protein, to provide high spatiotemporal resolution of mitotic phase. This approach visualizes cytokinesis and midbody formation as hallmarks of expansion of stem and somatic cells, and enables distinction from cell cycle variations. High-resolution microscopy in embryonic heart and brain tissues of enhanced green fluorescent protein–anillin transgenic mice allows live monitoring of cell division and quantitation of cell cycle kinetics. Analysis of cell division in hearts post injury shows that border zone cardiomyocytes in the infarct respond with increasing ploidy, but not cell division. Thus, the enhanced green fluorescent protein–anillin system enables monitoring and measurement of cell division in vivo and markedly simplifies in vitro analysis in fixed cells. The determination of cell proliferation and its distinction from incomplete cell cycle progression is often a critical element in cell biology and regenerative medicine. Current methods require uptake of bromodeoxyuridine or 3 H-thymidine, or immunostaining of fixed cells with cell cycle-specific antibodies. The former methods require complicated cellular uptake protocols for in vivo studies, and both methods poorly differentiate authentic cell division from endoreduplication, acytokinetic mitosis or DNA repair. Endoreduplication (DNA replication without karyokinesis or cytokinesis) and acytokinetic mitosis (karyokinesis without cytokinesis) occur during development and following injury in numerous cell types. To unequivocally identify proliferating cells in regenerative studies, double and triple stainings with separate cell cycle markers, such as Ki-67, pHH3 and Aurora-B kinase (AurB), are required; these techniques are technically challenging and subject to staining artefacts. These limitations often underlie controversies in the stem cell field regarding the occurrence of cell regeneration and the source of regenerative cells [1] , [2] , [3] . The late mitotic (M) phase of the cell cycle is accompanied by the assembly of a contractile ring, which forms at the cell cortex and constricts the cell membrane to form two daughter cells, and the midbody, which forms from the mitotic spindles just before abscission of the daughter cells. Thus, direct visualization of the contractile ring and the midbody is definitive proof of cell division and particularly important in muscle and other tissues in which prominent variations in the cell cycle must be distinguished from cell division. Moreover, visualization of the contractile ring and the midbody would enable determination of the cleavage furrow orientation, a key factor in the asymmetric division of neural stem cells, as cleavage orientation and inheritance of the apical midbody during embryonic development of neuroepithelium has been linked to subsequent cell fate [4] , [5] , [6] . Finally, observation of individual M-phase events in live cells would facilitate our understanding of the factors that govern cell fate decisions. Here we report the development of a system that allows direct visualization of these structures in live cells, by fusing enhanced green fluorescent protein (eGFP) to the scaffolding protein anillin, a component of the contractile ring that localizes to specific subcellular compartments during M-phase [7] . We demonstrate that eGFP–anillin enables visualization of M-phase cells in hearts and brains of transgenic mice and simplifies cytokinetic analysis of murine and human pluripotent cells. In addition, we also provide evidence that cardiomyocytes enter endocycles and become polyploid, but do not divide post-myocardial injury. eGFP–anillin expression marks proliferating cells We reasoned that the scaffolding protein anillin would constitute an ideal marker for cell division, as it is located in the nucleus during late G1-, S- and G2-phase of the cell cycle, in the cytoplasm and cell cortex in early M-phase, and in the contractile ring and midbody during and immediately upon cytokinesis ( Fig. 1a ). Following mitosis, anillin is ubiquitinated in early G1 by the anaphase-promoting complex associated to Cdh1 (APC Cdh1 ) and degraded by the proteasome. To visualize mitotic events, full-length mouse anillin protein was fused to the C-terminus of eGFP and placed under control of the ubiquitous CAG promoter ( Fig. 1a ). 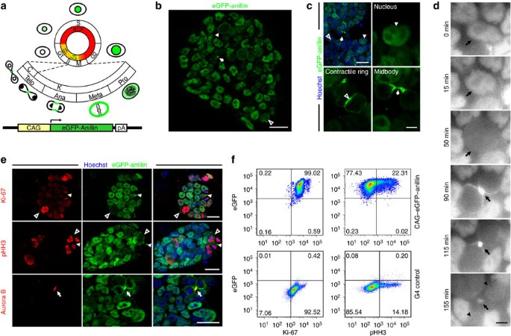Figure 1: eGFP–anillin expression is a mitotic marker in mouse pluripotent cells. (a) Schemes of subcellular localization of the eGFP–anillin fusion protein during the cell cycle and of the CAG–eGFP–anillin fusion construct: Anillin is fused to the C terminus of eGFP and its expression is under control of the CAG promoter. APC, anaphase-promoting complex; C, cytokinesis; Cdc20, cell-division cycle protein 20; Cdh1, Cdc20 homologue-1; K, karyokinesis; SCF, Skp, Cullin, F-box-containing complex. (b) Picture of a living colony of a stably transfected mESC line expressing eGFP–anillin under control of the CAG promoter. eGFP–anillin (green) localization in the cytoplasm (open arrowhead), cell cortex (solid arrowhead) and midbody (arrow). Scale bar, 25 μm. (c) Analysis of fixated transgenic mESCs; nuclei are stained with Hoechst nuclear dye (blue, upper left picture). Differential localization of eGFP–anillin (green) in the nucleus (solid arrowhead), cortex/contractile ring (open arrowhead) or midbody (arrow). Scale bars, 25 (upper left picture) and 5 μm (all other pictures). (d) Time-lapse images taken from a CAG–eGFP–anillin mESC clone. The arrows mark a cell with changing localization of the eGFP–anillin fluorescence signal during M-phase. The arrowheads point to the nuclei of the daughter cells. Scale bar, 5 μm. (e) Stainings for the proliferation markers Ki-67, pHH3 and Aurora-B kinase (all red) reveals co-labelling with the eGFP–anillin (green) fluorescence signal. Note localization in cytoplasm/cortex (open arrowheads), contractile rings (solid arrowheads) and midbodies (arrows); nuclei are stained with Hoechst dye (blue). Scale bar, 25 μm. (f) Flow-cytometric profiles of eGFP–anillin mESCs and non-transfected G4 mESCs stained for Ki-67 or pHH3, respectively. The majority of eGFP–anillin+cells is Ki-67+, a smaller fraction of eGFP–anillin+mESCs is positive for the M-phase marker pHH3. Figure 1: eGFP–anillin expression is a mitotic marker in mouse pluripotent cells. ( a ) Schemes of subcellular localization of the eGFP–anillin fusion protein during the cell cycle and of the CAG–eGFP–anillin fusion construct: Anillin is fused to the C terminus of eGFP and its expression is under control of the CAG promoter. APC, anaphase-promoting complex; C, cytokinesis; Cdc20, cell-division cycle protein 20; Cdh1, Cdc20 homologue-1; K, karyokinesis; SCF, Skp, Cullin, F-box-containing complex. ( b ) Picture of a living colony of a stably transfected mESC line expressing eGFP–anillin under control of the CAG promoter. eGFP–anillin (green) localization in the cytoplasm (open arrowhead), cell cortex (solid arrowhead) and midbody (arrow). Scale bar, 25 μm. ( c ) Analysis of fixated transgenic mESCs; nuclei are stained with Hoechst nuclear dye (blue, upper left picture). Differential localization of eGFP–anillin (green) in the nucleus (solid arrowhead), cortex/contractile ring (open arrowhead) or midbody (arrow). Scale bars, 25 (upper left picture) and 5 μm (all other pictures). ( d ) Time-lapse images taken from a CAG–eGFP–anillin mESC clone. The arrows mark a cell with changing localization of the eGFP–anillin fluorescence signal during M-phase. The arrowheads point to the nuclei of the daughter cells. Scale bar, 5 μm. ( e ) Stainings for the proliferation markers Ki-67, pHH3 and Aurora-B kinase (all red) reveals co-labelling with the eGFP–anillin (green) fluorescence signal. Note localization in cytoplasm/cortex (open arrowheads), contractile rings (solid arrowheads) and midbodies (arrows); nuclei are stained with Hoechst dye (blue). Scale bar, 25 μm. ( f ) Flow-cytometric profiles of eGFP–anillin mESCs and non-transfected G4 mESCs stained for Ki-67 or pHH3, respectively. The majority of eGFP–anillin + cells is Ki-67 + , a smaller fraction of eGFP–anillin + mESCs is positive for the M-phase marker pHH3. Full size image To demonstrate functionality of the eGFP–anillin fusion protein as a marker for cell division, we first generated stably transfected mouse embryonic stem cell (mESC) lines ( Supplementary Methods ). Live-cell imaging of eGFP fluorescence, as well as its analysis post-fixation in eGFP–anillin mESC colonies, revealed nuclear localization in the majority of cells (94.8±0.6% s.e.m. of n =4 mESC clones), and a subpopulation in which eGFP–anillin displayed cytoplasmatic/cortical (3.0±0.5%), contractile ring (0.9±0.1%) and midbody (1.4±0.0%) localization ( Fig. 1b,c , arrows; Fig. 1d ), as would be expected in continuously proliferating cells ( Fig. 1a ). We next examined whether the subcellular pattern of eGFP–anillin expression could distinguish specific cell cycle phases, by comparing eGFP expression with the expression of Ki-67 (marker for all cell cycle phases except G o ), pHH3 (marker for M-phase) and AurB (midbody marker; Fig. 1e ). Immunostainings for Ki-67, which lacks the cell cycle-specific subcellular localization of the eGFP–anillin signal, revealed a high overlap between Ki-67 + and eGFP–anillin + cells as analysed by microscopy (98.1%) and flow cytometry (99%; Fig. 1f ). The fraction of pHH3 + cells was significantly lower (24.4 and 22.2% when determined by microscopy and flow cytometry, respectively) than the fraction of Ki-67 + cells. Importantly, all pHH3 + cells were also eGFP–anillin + ( Fig. 1e,f ). Staining for AurB showed that eGFP–anillin localizes to the midbody after cytokinesis ( Fig. 1e ). These data were further supported by time-lapse microscopy, in which eGFP–anillin expression was detected in all proliferating cells. The expected M-phase distribution of the fusion protein in cytoplasm after nucleus dissolution was followed by localizaton in contractile rings and midbodies ( Supplementary Movie 1 ). To enable an even broader application of this system and to test its functionality in human cells, we generated a lentivirus ( Supplementary Methods ) and transduced human ESCs (H9) and human induced pluripotent stem cells (hiPSC); the virus consisted of the CAG–eGFP–anillin expression cassette in pSico, a well established second-generation lentiviral vector [8] ( Fig. 2a ). Approximately 15% of all hESCs and hiPSCs expressed eGFP–anillin and displayed complete overlap with Ki-67 staining ( Fig. 2b ). Nuclear and cytoplasmic localization of eGFP–anillin and localization in contractile rings or midbodies was observed ( Fig. 2b , arrows); pHH3 or AurB staining proved high cell cycle specificity of the eGFP signal ( Fig. 2b ). Expression of eGFP–anillin enabled measurement of M-subphase duration and of the complete cell cycle in individual hESCs and hiPSCs by live-cell imaging ( Fig. 2c ; Supplementary Movie 2 and Supplementary Methods ). In H9 hESCs, cell cycle duration was 17.0±0.5 h ( n =21), with an M-phase of 33±1 min and a brief early G1-phase of 26±3 min. 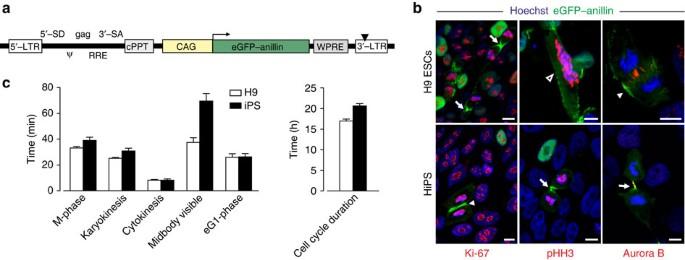Figure 2: eGFP–anillin marks proliferating cells in human iPS- and ES cell lines. (a) Scheme of the lentiviral vector: black triangle, mutation in 3′ LTR, leading to self inactivation (SIN vector); CAG, combination of early enhancer element of CMV (cytomegalovirus) promoter and chicken β-actin promoter; cPPT, central polypurine tract; eGFP-anillin, enhanced green fluorescent protein fused to anillin; gag, truncated group-specific antigen sequence; SA, splice acceptor sites; LTR, long terminal repeat; Psi, packaging signal; RRE, rev response element; SD, splice donor sites; WPRE, post-transcriptional regulatory element of woodchuck hepatitis virus. (b) Stainings of lentivirus CAG–eGFP–anillin-transduced human H9 ESCs and human iPS cells for the proliferation markers Ki-67, pHH3 and Aurora-B kinase (all three red). eGFP–anillin (green) has M-phase-specific localization in the nucleus, cytoplasm (open arrowhead), contractile ring (solid arrowhead) and midbodies (arrows); Ki-67 stains nucleoli in human cells; nuclei are stained with Hoechst dye (blue). Scale bars, 10 μm. (c) Analysis of cell cycle kinetics of human iPS and ESCs with time-lapse microscopy. Data are shown as mean±s.e.m. fromn=22 (iPS) andn=21 (H9) cells. Figure 2: eGFP–anillin marks proliferating cells in human iPS- and ES cell lines. ( a ) Scheme of the lentiviral vector: black triangle, mutation in 3′ LTR, leading to self inactivation (SIN vector); CAG, combination of early enhancer element of CMV (cytomegalovirus) promoter and chicken β-actin promoter; cPPT, central polypurine tract; eGFP-anillin, enhanced green fluorescent protein fused to anillin; gag, truncated group-specific antigen sequence; SA, splice acceptor sites; LTR, long terminal repeat; Psi, packaging signal; RRE, rev response element; SD, splice donor sites; WPRE, post-transcriptional regulatory element of woodchuck hepatitis virus. ( b ) Stainings of lentivirus CAG–eGFP–anillin-transduced human H9 ESCs and human iPS cells for the proliferation markers Ki-67, pHH3 and Aurora-B kinase (all three red). eGFP–anillin (green) has M-phase-specific localization in the nucleus, cytoplasm (open arrowhead), contractile ring (solid arrowhead) and midbodies (arrows); Ki-67 stains nucleoli in human cells; nuclei are stained with Hoechst dye (blue). Scale bars, 10 μm. ( c ) Analysis of cell cycle kinetics of human iPS and ESCs with time-lapse microscopy. Data are shown as mean±s.e.m. from n =22 (iPS) and n =21 (H9) cells. Full size image In summary, eGFP–anillin is a highly sensitive live cell marker of cell division in mouse and human pluripotent cells that discriminates individual cell cycle components, enabling quantitation of cell cycle kinetics of individual cells. eGFP–anillin is a proliferation marker in differentiating cells To assess our reporter system in somatic cells, we differentiated eGFP–anillin mESCs in embryoid bodies (EBs) and performed flow cytometric analysis of isolated cells. We found an excellent correlation between the eGFP–anillin signal and Ki-67 staining ( Fig. 3a ); as differentiation progressed, we observed a decrease in the percentage of eGFP–anillin + and Ki67 + cells ( Fig. 3a,b ) due to the increase in post-mitotic cells. Immunofluorescence staining of plated EBs ( Fig. 3c ) revealed a high overlap (93.3%, n =3 EBs of one ESC clone) of eGFP signals (50.7% of all cells) with Ki-67 staining (51.8% of all cells). Importantly, there was no accumulation of eGFP–anillin in non-cycling Ki-67 − cells ( Fig. 3c , arrows), most likely due to its proteasomal degradation by the activity of APC Cdh1 in post-mitotic cells. 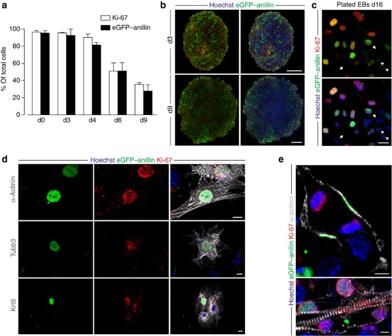Figure 3: eGFP–anillin is a mitotic marker in mESC-derived differentiating cells. (a) Percentage of Ki-67+and eGFP–anillin+cells in dissociated EBs at days 0 to 9 of differentiation; Ki-67 staining matches eGFP–anillin expression over the time course of differentiation. Data shown are mean±range of one differentiation experiment withn=2 orn=3 (day 4) different eGFP–anillin mESC clones. (b) Sections of transgenic murine eGFP–anillin EBs after 3 and 9 days of differentiation. On day 3, eGFP–anillin+(green) cells are found throughout the EB; at day 9, proliferation is restricted to the cortical areas of the EB; nuclei are stained with Hoechst dye (blue). Scale bar, 200 μm. (c) Staining for Ki-67 (red) of plated EBs at day 16 of differentiation revealed a high overlap with eGFP–anillin (green) expression; Ki-67−and eGFP–anillin−cells are marked by arrows. Note that some of the weak eGFP–anillin+cells have a very faint, but visible Ki-67 signal (arrowheads); nuclei are stained with Hoechst nuclear dye (blue). Scale bar, 25 μm. (d) EB-derived cells (day 12 of differentiation, 2 days after plating) from an eGFP–anillin mESC line are isolated and stained with subtype-specific markers: α-actinin for mesodermal, Tubb3 for neuroectodermal, and Krt8 for endodermal cells (all white). eGFP–anillin+cells (green) co-stain for Ki-67 (red); nuclei are stained with Hoechst nuclear dye (blue). Scale bars, 10 μm. (e) eGFP–anillin (green) fluorescence marked proliferating cardiomyocytes due to its specific position in contractile rings and midbodies; the cells are identified as cardiomyocytes based on α-actinin+staining (white) and co-labelled with Ki-67 (red); nuclei are stained with Hoechst dye (blue). Scale bars, 5 μm. Figure 3: eGFP–anillin is a mitotic marker in mESC-derived differentiating cells. ( a ) Percentage of Ki-67 + and eGFP–anillin + cells in dissociated EBs at days 0 to 9 of differentiation; Ki-67 staining matches eGFP–anillin expression over the time course of differentiation. Data shown are mean±range of one differentiation experiment with n =2 or n =3 (day 4) different eGFP–anillin mESC clones. ( b ) Sections of transgenic murine eGFP–anillin EBs after 3 and 9 days of differentiation. On day 3, eGFP–anillin + (green) cells are found throughout the EB; at day 9, proliferation is restricted to the cortical areas of the EB; nuclei are stained with Hoechst dye (blue). Scale bar, 200 μm. ( c ) Staining for Ki-67 (red) of plated EBs at day 16 of differentiation revealed a high overlap with eGFP–anillin (green) expression; Ki-67 − and eGFP–anillin − cells are marked by arrows. Note that some of the weak eGFP–anillin + cells have a very faint, but visible Ki-67 signal (arrowheads); nuclei are stained with Hoechst nuclear dye (blue). Scale bar, 25 μm. ( d ) EB-derived cells (day 12 of differentiation, 2 days after plating) from an eGFP–anillin mESC line are isolated and stained with subtype-specific markers: α-actinin for mesodermal, Tubb3 for neuroectodermal, and Krt8 for endodermal cells (all white). eGFP–anillin + cells (green) co-stain for Ki-67 (red); nuclei are stained with Hoechst nuclear dye (blue). Scale bars, 10 μm. ( e ) eGFP–anillin (green) fluorescence marked proliferating cardiomyocytes due to its specific position in contractile rings and midbodies; the cells are identified as cardiomyocytes based on α-actinin + staining (white) and co-labelled with Ki-67 (red); nuclei are stained with Hoechst dye (blue). Scale bars, 5 μm. Full size image We next investigated whether the eGFP–anillin construct marked cycling, mESC-derived cells of all three germ layers ( Fig. 3d ). This was the case, as eGFP–anillin + cells of the mesodermal (α-actinin + ), neuroectodermal (Tubb3 + ) and endodermal lineage (Krt8 + ) were observed; the specificity of the eGFP–anillin signal was confirmed by Ki-67 + staining. In EB-derived cardiomyocytes, eGFP–anillin expression was observed not only in the nuclei, but also in contractile rings and midbodies ( Fig. 3e ). Dividing cardiomyocytes displayed a loss of cross-striated structures, as previously reported [9] . eGFP–anillin + cardiomyocytes were also Ki-67 + , indicating that these cells were in the cell cycle, but Ki-67 expression could not distinguish between dividing cells and those undergoing merely cell cycle activity such as DNA synthesis. Conversely, the presence of an eGFP–anillin + midbody unequivocally identified cardiomyocytes that had just separated, discriminating these cells from those undergoing endoduplication or acytokinetic mitosis. To unequivocally show that the eGFP–anillin system is able to distinguish between cell division and incomplete cell cycle progression, we used trophoblast stem (TS) cells. These cells are known to rapidly proliferate in the undifferentiated state, but to undergo endoreduplication upon differentiation to trophoblast giant cells (TGCs) [10] . TS cells were transiently transfected with an eGFP–anillin expression construct and differentiated by withdrawal of FGF4 and addition of Cdk1 inhibitor [11] ( Supplementary Methods ). Our experiments revealed that eGFP–anillin localized to contractile rings and midbodies in undifferentiated TS cells ( Fig. 4a arrowhead). In contrast, differentiation of TS cells led to almost exclusive nuclear localization of eGFP–anillin within 4 h ( Fig. 4a ); differentiating TS cells changed morphologically into TGCs ( Fig. 4a , dotted line). This was underscored by the typical increase in DNA content up to 16C, as measured by Hoechst staining ( Fig. 4b ), and cell size ( Fig. 4c ). Within 48 h, the majority of TS cells had adopted a TGC fate with large eGFP–anillin + nuclei ( Fig. 4a , dotted line). We also determined the specific sub-phases of the endocycle in which eGFP–anillin was expressed. For this purpose, cells were stained against cyclin A and p57 Kip2 known markers of endo S-phase and endo G2-phase, respectively [12] . Nuclear eGFP–anillin signals were found to colocalize with cyclin A ( Fig. 4d ), but not with p57 ( Fig. 4d arrows), proving that eGFP–anillin marks TGCs in S-phase. 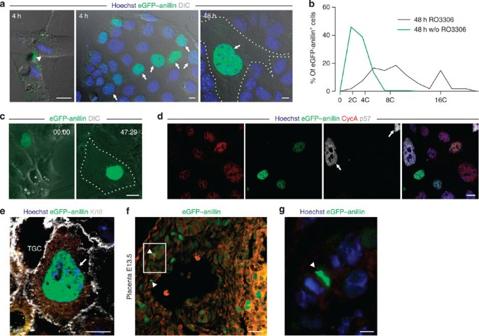Figure 4: The eGFP–anillin system distinguishes between cell division and endoreduplication in TS cells. (a) Epifluorescence pictures of eGFP–anillin-transfected TS cells 4 (upper and lower left pictures) and 48 h (lower right picture) after addition of RO3306. eGFP–anillin (green) is localized in the midbody of undifferentiated TS cells (arrowhead), but in the nucleus of differentiating, endoreduplicating TS cells (arrows). After 48 h of differentiation, typical TGCs (dotted line in DIC overlay) with nuclear eGFP–anillin localization can be observed; nuclei are stained with Hoechst nuclear dye (blue). Scale bars, 10 μm. (b) Percentage of distribution of nuclear DNA content of TS cells without (green line,n=200) or 48 h after addition of RO3306 (black line,n=54).C=C-value. (c) Time-lapse images taken from a differentiating TGC (dotted line in DIC image) expressing eGFP–anillin (green) at 0 and 47:30 h of differentiation. Scale bar, 20 μm. (d) Stainings of differentiating TGCs transfected with eGFP–anillin for cyclin A (red) and p57Kip2(white). The eGFP–anillin signal (green) co-localizes with cyclin A, but not p57 (arrows); nuclei are stained with Hoechst nuclear dye (blue). Scale bar, 20 μm. (e) TGC in placenta of transgenic mice display exclusively nuclear eGFP–anillin localization (green, TGC, arrow). Scale bar, 25 μm. (f) Chorionic plate of an E13.5 eGFP–anillin placenta. M-phase typical localizations of eGFP (arrowheads) are seen. White box illustrates the area shown ing; autofluorescence is red. Scale bar, 25 μm. (g) Chorionic plate cell with eGFP–anillin (green) localization to the contractile ring. Nuclei are stained blue; scale bar, 5 μm. Figure 4: The eGFP–anillin system distinguishes between cell division and endoreduplication in TS cells. ( a ) Epifluorescence pictures of eGFP–anillin-transfected TS cells 4 (upper and lower left pictures) and 48 h (lower right picture) after addition of RO3306. eGFP–anillin (green) is localized in the midbody of undifferentiated TS cells (arrowhead), but in the nucleus of differentiating, endoreduplicating TS cells (arrows). After 48 h of differentiation, typical TGCs (dotted line in DIC overlay) with nuclear eGFP–anillin localization can be observed; nuclei are stained with Hoechst nuclear dye (blue). Scale bars, 10 μm. ( b ) Percentage of distribution of nuclear DNA content of TS cells without (green line, n =200) or 48 h after addition of RO3306 (black line, n =54). C = C -value. ( c ) Time-lapse images taken from a differentiating TGC (dotted line in DIC image) expressing eGFP–anillin (green) at 0 and 47:30 h of differentiation. Scale bar, 20 μm. ( d ) Stainings of differentiating TGCs transfected with eGFP–anillin for cyclin A (red) and p57 Kip2 (white). The eGFP–anillin signal (green) co-localizes with cyclin A, but not p57 (arrows); nuclei are stained with Hoechst nuclear dye (blue). Scale bar, 20 μm. ( e ) TGC in placenta of transgenic mice display exclusively nuclear eGFP–anillin localization (green, TGC, arrow). Scale bar, 25 μm. ( f ) Chorionic plate of an E13.5 eGFP–anillin placenta. M-phase typical localizations of eGFP (arrowheads) are seen. White box illustrates the area shown in g ; autofluorescence is red. Scale bar, 25 μm. ( g ) Chorionic plate cell with eGFP–anillin (green) localization to the contractile ring. Nuclei are stained blue; scale bar, 5 μm. Full size image Time-lapse microscopy illustrated a fluctuation of the eGFP–anillin signal in nuclei of TGCs. eGFP–anillin was visible during the endo S-phase and degraded during endo G-phase ( Supplementary Movie 3 ), whereas in undifferentiated TS cells, cell division with formation of eGFP–anillin + contractile rings and midbodies occured ( Fig. 4a ; Supplementary Movie 4 ). These data enabled us to directly quantify the duration of the endocycle yielding 25.3±2.7 h ( n =14), of the endo G-phase with 12.6±2.2 h and of the endo S phase with 14.8±1.6 h, respectively; these data are in agreement with indirect measurements of cell cycle duration [11] . Thus, our experiments demonstrate that expression of eGFP–anillin in midbodies identifies cells in the final stages of cytokinesis, enabling easy and accurate identification of dividing cells versus cells with atypical cell cycle progression in live cell experiments. Establishing transgenic eGFP–anillin mouse lines To evaluate the feasibility of eGFP–anillin as a proliferation marker in vivo , we generated two transgenic mouse lines expressing eGFP–anillin under control of the CAG promoter, by aggregation of eGFP–anillin mESCs with wild-type tetraploid embryos ( Supplementary Methods ). To show that the system discriminates between cell division and endoreduplication in the transgenic mouse model, we examined TGCs in analogy to our in vitro experiments. As expected, eGFP–anillin signals were localized exclusively in the nuclei ( Fig. 4e , arrow) of these endoreduplicating cells, indicating the absence of the anillin-containing structures present during cytokinesis. By contrast, in dividing cells of the chorionic plate, eGFP–anillin was found in contractile rings and midbodies ( Fig. 4f,g , arrowheads). Dissection of embryos from eGFP–anillin mice at E10.5 revealed eGFP–anillin expression in all tissues ( Fig. 5a ), but strongest signals were observed in hearts ( Fig. 5b , dotted square). Staining for Ki-67 in embryonic and neonatal (E10.5, E18.5, P3) hearts revealed good (>90% for E18.5) overlap with eGFP–anillin expression in atria and ventricles ( Fig. 5c–f ). To facilitate the identification of cardiomyocytes without additional immunostaining, eGFP–anillin mice were crossed with a transgenic mouse line expressing the red fluorescence protein mCherry under control of the cardiac-specific αMHC promoter ( Fig. 5g , arrows). Importantly, eGFP–anillin was observed in contractile rings and midbodies of mCherry + cardiomyocytes at E13.5 ( Fig. 5g , arrowheads), and of α-actinin + cardiomyocytes at E18.5 ( Fig. 5e ). 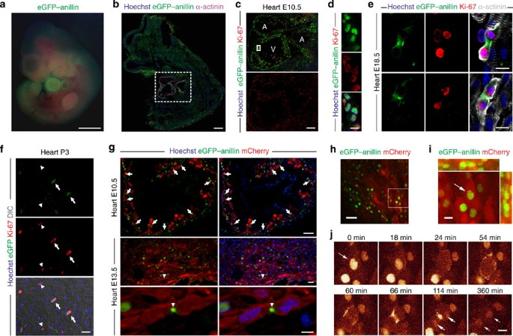Figure 5: eGFP–anillin is a mitotic markerin vivoduring embryonic development. (a) Epifluorescence picture taken from an E10.5 eGFP–anillin transgenic embryo showing eGFP fluorescence (green); autofluorescence is red. Scale bar, 1 mm. (b) Sagittal sections of an E10.5 eGFP–anillin embryo reveals eGFP expression (green) in all tissues; cardiomyocytes are identified by α-actinin staining (magenta, dashed square). Scale bar, 200 μm. (c) Sagittal sections through an E10.5 eGFP–anillin heart evidence that atria (A) and ventricle (V) are strongly eGFP–anillin+(green). Ki-67 staining (red) of same section proves overlap between both fluorescence signals; nuclei are blue in the merged image. Scale bar, 100 μm, (d) Magnification of boxed area inc. Ventricular cardiomyocytes display eGFP–anillin (green) expression and are Ki-67+(red); nuclei are blue in the merged image. Scale bar, 10 μm. (e) Proliferating α-actinin+(white) cardiomyocytes in sections from an E18.5 eGFP–anillin heart are identified by eGFP labelling (green) of contractile rings or midbodies; Ki-67 staining is red; nuclei are blue. Scale bar, 10 μm. (f) Co-stainings for eGFP (green) and Ki-67 (red) in cross sections of a P3 eGFP–anillin+heart reveal restriction of the eGFP signal to cardiomyocytes (arrows). Arrowheads mark Ki-67+/eGFP−cells; nuclei are blue. Scale bar, 25 μm. (g) Sections of E10.5 and E13.5 hearts from eGFP–anillin/αMHC–mCherry mice. Proliferating cardiomyocytes (arrows) are identified by co-expression of mCherry (red) and eGFP–anillin (green). Scale bars, 50 (E10.5), 20 and 5 μm (E13.5). (h) Optical section from an eGFP–anillin/αMHC–mCherry E11.5 heart showing eGFP–anillin+(green) and mCherry+(red) cells. The white box illustrates the area shown iniandj. Scale bar, 40 μm. (i) The eGFP–anillin+nucleus (arrow) can be attributed to a αMHC–mCherry+cell. The illustrated single optical section (x,y) is located in the centre of 13 planes. The corresponding x- (top) and y-projections (right) are given. Scale bar, 10 μm. (j) Time series of the same individual myocyte (white arrow incand att=0) imaged without optical filtering. A complete M-phase is visualized based on eGFP–anillin fluorescence during 6 h. Two nuclei of daughter cells become visible starting at 114 min (white arrows). Scale bar, 10 μm. Figure 5: eGFP–anillin is a mitotic marker in vivo during embryonic development. ( a ) Epifluorescence picture taken from an E10.5 eGFP–anillin transgenic embryo showing eGFP fluorescence (green); autofluorescence is red. Scale bar, 1 mm. ( b ) Sagittal sections of an E10.5 eGFP–anillin embryo reveals eGFP expression (green) in all tissues; cardiomyocytes are identified by α-actinin staining (magenta, dashed square). Scale bar, 200 μm. ( c ) Sagittal sections through an E10.5 eGFP–anillin heart evidence that atria (A) and ventricle (V) are strongly eGFP–anillin + (green). Ki-67 staining (red) of same section proves overlap between both fluorescence signals; nuclei are blue in the merged image. Scale bar, 100 μm, ( d ) Magnification of boxed area in c . Ventricular cardiomyocytes display eGFP–anillin (green) expression and are Ki-67 + (red); nuclei are blue in the merged image. Scale bar, 10 μm. ( e ) Proliferating α-actinin + (white) cardiomyocytes in sections from an E18.5 eGFP–anillin heart are identified by eGFP labelling (green) of contractile rings or midbodies; Ki-67 staining is red; nuclei are blue. Scale bar, 10 μm. ( f ) Co-stainings for eGFP (green) and Ki-67 (red) in cross sections of a P3 eGFP–anillin + heart reveal restriction of the eGFP signal to cardiomyocytes (arrows). Arrowheads mark Ki-67 + /eGFP − cells; nuclei are blue. Scale bar, 25 μm. ( g ) Sections of E10.5 and E13.5 hearts from eGFP–anillin/αMHC–mCherry mice. Proliferating cardiomyocytes (arrows) are identified by co-expression of mCherry (red) and eGFP–anillin (green). Scale bars, 50 (E10.5), 20 and 5 μm (E13.5). ( h ) Optical section from an eGFP–anillin/αMHC–mCherry E11.5 heart showing eGFP–anillin + (green) and mCherry + (red) cells. The white box illustrates the area shown in i and j . Scale bar, 40 μm. ( i ) The eGFP–anillin + nucleus (arrow) can be attributed to a αMHC–mCherry + cell. The illustrated single optical section (x,y) is located in the centre of 13 planes. The corresponding x- (top) and y-projections (right) are given. Scale bar, 10 μm. ( j ) Time series of the same individual myocyte (white arrow in c and at t =0) imaged without optical filtering. A complete M-phase is visualized based on eGFP–anillin fluorescence during 6 h. Two nuclei of daughter cells become visible starting at 114 min (white arrows). Scale bar, 10 μm. Full size image Although the numbers of embryonic cardiomyocytes in different cell cycle phases have been characterized over the course of heart growth [13] , the overall cell cycle length and duration of individual sub-phases are still unknown. We determined durations of key cell cycle phases using two-photon imaging of individual cells in E11.5 hearts collected from double transgenic mice. Ventricular cardiomyocytes with cell cycle activity were identified based on cytoplasmic mCherry- and nuclear eGFP–anillin expression, respectively ( Fig. 5h,i ). In cardiomyocytes, we observed nuclear dissolution, formation and contraction of the contractile ring, midbody formation and re-expression of eGFP–anillin in the nuclei of the newly formed daughter cells at high spatial resolution ( Fig. 5j and Supplementary Movie 5 ). M-phase duration was 79±19 min ( n =3), whereas early G1-phase was 27±5 min; contractile rings persisted for 26±5 min and midbodies for 86±18 min. This prolonged expression of eGFP–anillin in the midbody enabled identification of cardiomyocytes that had proliferated, even post cell division. Similarly, M-phase and cell division were monitored in other non-cardiomyocytes within the heart ( Supplementary Movie 6 ), most of which displayed a fibroblast-like morphology. Midbodies persisted in these cells even longer (101±17 min), whereas M-phase (72±2 min, n =7) and early G1-phase were comparable (29±5 min) to cardiomyocytes. eGFP–anillin marks proliferation of neural progenitors We explored eGFP–anillin expression in the embryonic brain, as such studies could provide new insights into brain development. During early neurogenesis (E10.5), eGFP–anillin was detected in nuclei and midbodies in the apical region of the ventricular zone (VZ) of the neuroepithelium ( Fig. 6a , arrows), indicating cellular expansion. Similarly, eGFP–anillin expression was apparent during mid-neurogenesis (E14.5) in the dorsal telencephalon, the period of peak progenitor heterogeneity in this region. Nuclear signals were clearly visible in both proliferative regions of the forebrain, namely the VZ and the sub-VZ (SVZ; Fig. 6b ). The strongest expression was found in nuclei of radial glia (RG) cells in the apical region of the VZ, which are known to be highly proliferative at this stage. Conversely, between this region and the SVZ, we noted fewer eGFP–anillin + nuclei, reflecting the presence of apical progenitor cells in G1-phase of the cell cycle, which are eGFP–anillin − ( Fig. 6b ). Besides the typical localization of mitotic nuclei, the specificity of the eGFP–anillin signal in the neuroepithelium was also corroborated by Ki-67 and Tubb3 co-stainings. Tubb3 is mostly contained in differentiating neurons and their processes ( Fig. 6b ), and at this stage, these cells are preferentially located in the neuronal layer and the intermediate zone, through which many neurons migrate on their way to the neuronal layer ( Fig. 6b , IZ). Tubb3 + neurons were eGFP–anillin − and Ki-67 − , indicating a post-mitotic status ( Fig. 6b,c ). Also in the SVZ, where proliferative basal progenitor (BP) cells reside, eGFP–anillin + nuclei were Ki-67 + and Tubb3 − ( Fig. 6b,c ). To examine further the progenitor sub-types, we identified the proliferative RG and BP cells with the specific antigens brain lipid-binding protein (BLBP; Fig. 6d ) and Tbr2 ( Fig. 6e ), respectively. Co-staining for eGFP–anillin with an eGFP antibody revealed a high overlap with RG and BP cells. 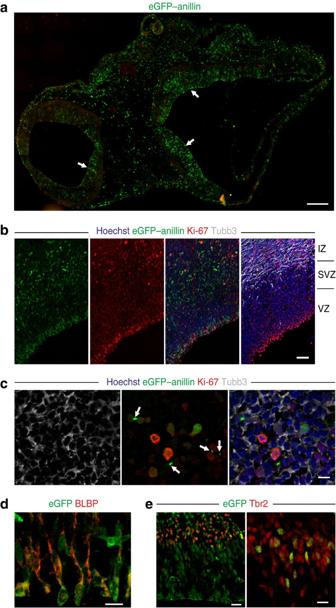Figure 6: eGFP–anillin specifically marks proliferating radial glia (RG) and basal progenitor (BP) cells at mid neurogenesis. (a) Cross sections through the brain of an E10.5 fixed embryo show eGFP–anillin signals in the neuroepithelium (arrows). Scale bar, 200 μm. (b) Cross section of E14.5 cerebral cortex from eGFP–anillin mice immunostained for Ki-67 (red), Tubb3 (white) and Hoechst (blue). Notice overlap of Ki-67 and eGFP–anillin (green) fluorescence in the merged image and loss of proliferative marker Ki-67 in differentiated neurons (Tubb3). IZ=intermediate zone, SVZ=subventricular zone, VZ=ventricular zone. Scale bar, 50 μm. (c) eGFP–anillin+midbodies and contractile rings indicative for cell division are observed in neuroepithelial (arrows) but not Tubb3+(white) cells. Ki-67 staining (red) correlates with eGFP–anillin expression (green). Nuclei are stained with Hoechst dye (blue). Scale bar, 10 μm. (d) At E14.5 eGFP staining co-localizes with brain lipid-binding protein (BLBP; red), a known marker for RG cells in the VZ (single optical section). Scale bar, 10 μm. (e) BP cells of the cortical SVZ from eGFP–anillin mice co-stain for eGFP and the transcription factor Tbr2, a marker for BPs (red). Scale bar, 10 μm. Figure 6: eGFP–anillin specifically marks proliferating radial glia (RG) and basal progenitor (BP) cells at mid neurogenesis. ( a ) Cross sections through the brain of an E10.5 fixed embryo show eGFP–anillin signals in the neuroepithelium (arrows). Scale bar, 200 μm. ( b ) Cross section of E14.5 cerebral cortex from eGFP–anillin mice immunostained for Ki-67 (red), Tubb3 (white) and Hoechst (blue). Notice overlap of Ki-67 and eGFP–anillin (green) fluorescence in the merged image and loss of proliferative marker Ki-67 in differentiated neurons (Tubb3). IZ=intermediate zone, SVZ=subventricular zone, VZ=ventricular zone. Scale bar, 50 μm. ( c ) eGFP–anillin + midbodies and contractile rings indicative for cell division are observed in neuroepithelial (arrows) but not Tubb3 + (white) cells. Ki-67 staining (red) correlates with eGFP–anillin expression (green). Nuclei are stained with Hoechst dye (blue). Scale bar, 10 μm. ( d ) At E14.5 eGFP staining co-localizes with brain lipid-binding protein (BLBP; red), a known marker for RG cells in the VZ (single optical section). Scale bar, 10 μm. ( e ) BP cells of the cortical SVZ from eGFP–anillin mice co-stain for eGFP and the transcription factor Tbr2, a marker for BPs (red). Scale bar, 10 μm. Full size image Next we determined M-phase-specific localization of eGFP–anillin as a bona fide marker of cell division, correlating its expression with that of p-vimentin ( Fig. 7a ) and pHH3 ( Fig. 7b ). eGFP–anillin localized to the cell cortex, cleavage furrow and midbodies of apical progenitor cells, which were also pHH3 + , p-vimentin + or Ki-67 + ( Fig. 7a–c ). The eGFP–anillin system also enabled resolution of the spatiotemporal events and dynamics of cell division in apical progenitor cells and BP cells in time-lapse confocal imaging of acute brain slices. Imaging individual nuclei of apical progenitor cells revealed basal to apical movement of the cell body ( Fig. 7d , white arrow), the so-called interkinetic nuclear migration. We could also visualize the division of the basal process of RG cells, which takes place before the division of the cell body ( Supplementary Movie 7 ) and the subsequent unidirectional ingression of the perpendicular cleavage furrow ( Fig. 7d , red arrow). In contrast to RG cells, dividing BP cells remained located in the SVZ ( Fig. 7d , yellow arrow, and Supplementary Movie 8 ) and displayed bidirectional ingression of a non-perpendicular cleavage furrow ( Fig. 7d ; Supplementary Movie 8 ). Duration of M-phase in RG cells was 47±5 min in these experiments. 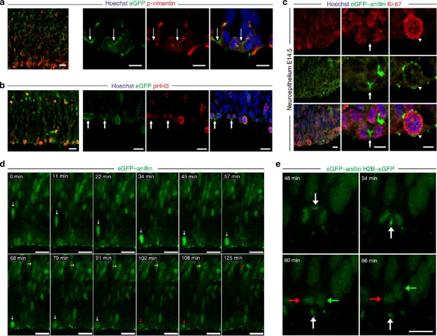Figure 7: eGFP–anillin enables live monitoring of neural progenitor cell division in acute brain slices. (a,b) Cross sections of the cerebral cortex of an E14.5 embryo reveal co-staining for anti-eGFP and anti-p-vimentin or anti-pHH3 in the neuroepithelium. Close-ups of stainings of apical progenitor cells for pHH3 and p-vimentin (both red), identifies cells in M-phase. eGFP–anillin+contractile rings and midbodies are clearly visible (arrows). Nuclei are stained with Hoechst dye (blue). Scale bars, 5 (a) and 10 μm (b). (c) Cross section of the cerebral cortex of an E14.5 embryo shows eGFP–anillin expression (green) in the neuroepithelium and co-localization with Ki-67 staining (red). Close-ups depict apical progenitor cells, these are Ki-67+(red) and eGFP–anillin is detected in contractile rings (arrows) or in cortical/cytoplasmatic localization (arrowheads), proving different stages of M-phase. Nuclei are stained with Hoechst dye (blue). Scale bars, 5 μm. (d) Time-lapse images taken from an acute brain slice of an E14.5 eGFP–anillin embryo. Representative apical (white arrow) and basal (yellow arrow) progenitor cells are shown. Formation of contractile rings is indicated by red arrows. Scale bar, 20 μm. (e) Time-lapse images from an acute brain slice of an E14.5 eGFP–anillin/CAG–H2B–eGFP double transgenic embryo with nuclear H2B–eGFP signal in all cells. The eGFP–anillin signal becomes bright green and markedly visible during cytokinesis and formation of the midbody (white arrows). After cell division, the midbody remains close to the cell body of one daughter cell (red arrows), whereas the cell body of the other daughter cell migrates towards the basal side of the neuroepithelium (green arrows), possibly indicating asymmetry in inheritance of the midbody. Scale bar, 10 μm. Figure 7: eGFP–anillin enables live monitoring of neural progenitor cell division in acute brain slices. ( a , b ) Cross sections of the cerebral cortex of an E14.5 embryo reveal co-staining for anti-eGFP and anti-p-vimentin or anti-pHH3 in the neuroepithelium. Close-ups of stainings of apical progenitor cells for pHH3 and p-vimentin (both red), identifies cells in M-phase. eGFP–anillin + contractile rings and midbodies are clearly visible (arrows). Nuclei are stained with Hoechst dye (blue). Scale bars, 5 ( a ) and 10 μm ( b ). ( c ) Cross section of the cerebral cortex of an E14.5 embryo shows eGFP–anillin expression (green) in the neuroepithelium and co-localization with Ki-67 staining (red). Close-ups depict apical progenitor cells, these are Ki-67 + (red) and eGFP–anillin is detected in contractile rings (arrows) or in cortical/cytoplasmatic localization (arrowheads), proving different stages of M-phase. Nuclei are stained with Hoechst dye (blue). Scale bars, 5 μm. ( d ) Time-lapse images taken from an acute brain slice of an E14.5 eGFP–anillin embryo. Representative apical (white arrow) and basal (yellow arrow) progenitor cells are shown. Formation of contractile rings is indicated by red arrows. Scale bar, 20 μm. ( e ) Time-lapse images from an acute brain slice of an E14.5 eGFP–anillin/CAG–H2B–eGFP double transgenic embryo with nuclear H2B–eGFP signal in all cells. The eGFP–anillin signal becomes bright green and markedly visible during cytokinesis and formation of the midbody (white arrows). After cell division, the midbody remains close to the cell body of one daughter cell (red arrows), whereas the cell body of the other daughter cell migrates towards the basal side of the neuroepithelium (green arrows), possibly indicating asymmetry in inheritance of the midbody. Scale bar, 10 μm. Full size image We also monitored daughter cells following cell division after degradation of eGFP–anillin, by crossing eGFP–anillin mice with the H2B–eGFP mouse line, in which eGFP is constitutively expressed in the nuclei [14] . The localized eGFP–anillin signal enabled determination of the inheritance of the midbody of apical progenitors by confocal time-lapse imaging ( Fig. 7e ; Supplementary Movie 9 ). Interestingly, and in contrast to analysis performed at earlier embryonic stages [5] , midbody release of apical progenitor cells into the ventricular lumen after division could not be observed at the stages analysed (E14–E15). Analysis of cardiac regeneration post injury Adult CAG–eGFP–anillin mice do not express eGFP–anillin in cardiac muscle ( Fig. 8a ) because of the known low rate of proliferation of cardiac muscle cells and the permanent activity of the APC Cdh1 [15] . The degree of post-injury cardiac regeneration remains controversial [16] ; therefore, CAG–eGFP–anillin mice were used to re-assess repair following cryoinjury and left coronary artery ligation (left anterior descending (LAD)) [17] . At day 4 after lesion (d4), we detected a large population of eGFP–anillin-expressing cells ( Fig. 8b ), which were distributed throughout the lesion (infarcted area) and to a lesser extent in the border zone (BZ), but not in intact myocardium. Most of these cells were identified as myofibroblasts by α-smooth muscle actin + staining ( Fig. 8c , arrows). In some of these cells (8.1%), eGFP–anillin was located in the contractile ring or midbody ( Fig. 8c , arrowhead and open arrowhead), proving ongoing cell division. 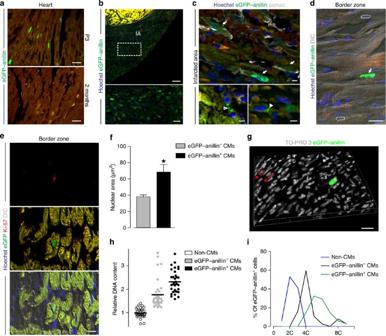Figure 8: Transgenic eGFP–anillin mice reveal endoreduplication in cardiomyocytes after cardiac injury. (a) eGFP–anillin expression (green) can be observed in cardiomyocytes of P3 mice; in 2-month-old mice, no eGFP–anillin signals can be detected in the heart. Scale bar, 25 μm. (b) Sections through a heart of an adult eGFP–anillin transgenic mouse 4 days after cryoinfarction (CI). eGFP–anillin fluorescence (green) reveals numerous proliferating cells in the infarcted area (IA); the myocardium adjacent to the lesion is identified based on its strong autofluorescence (yellow, BZ (border zone)); nuclei are stained with Hoechst dye (blue). Scale bars, 100 (overview) and 25 μm (magnification). (c) Positive staining for asmac (white) identifies the eGFP–anillin-expressing cells (green) as myofibroblasts (arrows). High magnification of such cells reveals eGFP–anillin localization in contractile rings (open arrowhead) and midbodies (solid arrowhead) proving cell division; nuclei are blue; autofluorescence is red. Scale bars, 5 μm. (d) Some of the cardiomyocytes in the BZ (LAD d12) show nuclear localization of eGFP–anillin (green, arrow); none displays a contractile ring or midbody. Nuclei of eGFP–anillin−cardiomyocytes (white dotted lines) are blue. Scale bar, 20 μm. (e) Co-stainings of cardiomyocytes against eGFP and Ki-67 in the BZ of the lesion revealed double-positive nuclei; scale bar, 10 μm. (f) Quantitation of nuclear area of cardiomyocytes in the BZ of d12CI and LAD hearts reveals that eGFP–anillin+nuclei (n=13 hearts) are significantly larger than eGFP–anillin−nuclei (n=6 hearts). Data are shown as mean±s.e.m., *P<0.05 (Student'st-test). (g) Three-dimensional (3D) confocal reconstruction of a 50-μm section from a d12 CI heart displaying an eGFP–anillin+nucleus (green) in a BZ cardiomyocyte, Two nuclei of eGFP–anillin−cardiomyocytes are shown (red arrows and red dotted lines). Nuclei are stained with TO-PRO 3 iodide (white). Scale bar, 20 μm. (h) Scatter plot showing mean DNA content of eGFP–anillin+cardiomyocytes (n=33), eGFP–anillin−cardiomyocytes (n=37) and non-cardiomyocytes (PECAM+endothelial cells,n=33) from sections (n=6) of a d12 CI heart (n=1). (i) Percentage of distribution of nuclear DNA content in eGFP–anillin+cardiomyocytes (green line,n=33), eGFP–anillin−cardiomyocytes (black line,n=37) and endothelial cells (blue line,n=33).C=C-value. Figure 8: Transgenic eGFP–anillin mice reveal endoreduplication in cardiomyocytes after cardiac injury. ( a ) eGFP–anillin expression (green) can be observed in cardiomyocytes of P3 mice; in 2-month-old mice, no eGFP–anillin signals can be detected in the heart. Scale bar, 25 μm. ( b ) Sections through a heart of an adult eGFP–anillin transgenic mouse 4 days after cryoinfarction (CI). eGFP–anillin fluorescence (green) reveals numerous proliferating cells in the infarcted area (IA); the myocardium adjacent to the lesion is identified based on its strong autofluorescence (yellow, BZ (border zone)); nuclei are stained with Hoechst dye (blue). Scale bars, 100 (overview) and 25 μm (magnification). ( c ) Positive staining for asmac (white) identifies the eGFP–anillin-expressing cells (green) as myofibroblasts (arrows). High magnification of such cells reveals eGFP–anillin localization in contractile rings (open arrowhead) and midbodies (solid arrowhead) proving cell division; nuclei are blue; autofluorescence is red. Scale bars, 5 μm. ( d ) Some of the cardiomyocytes in the BZ (LAD d12) show nuclear localization of eGFP–anillin (green, arrow); none displays a contractile ring or midbody. Nuclei of eGFP–anillin − cardiomyocytes (white dotted lines) are blue. Scale bar, 20 μm. ( e ) Co-stainings of cardiomyocytes against eGFP and Ki-67 in the BZ of the lesion revealed double-positive nuclei; scale bar, 10 μm. ( f ) Quantitation of nuclear area of cardiomyocytes in the BZ of d12CI and LAD hearts reveals that eGFP–anillin + nuclei ( n =13 hearts) are significantly larger than eGFP–anillin − nuclei ( n =6 hearts). Data are shown as mean±s.e.m., * P <0.05 (Student's t -test). ( g ) Three-dimensional (3D) confocal reconstruction of a 50-μm section from a d12 CI heart displaying an eGFP–anillin + nucleus (green) in a BZ cardiomyocyte, Two nuclei of eGFP–anillin − cardiomyocytes are shown (red arrows and red dotted lines). Nuclei are stained with TO-PRO 3 iodide (white). Scale bar, 20 μm. ( h ) Scatter plot showing mean DNA content of eGFP–anillin + cardiomyocytes ( n =33), eGFP–anillin − cardiomyocytes ( n =37) and non-cardiomyocytes (PECAM + endothelial cells, n =33) from sections ( n =6) of a d12 CI heart ( n =1). ( i ) Percentage of distribution of nuclear DNA content in eGFP–anillin + cardiomyocytes (green line, n =33), eGFP–anillin − cardiomyocytes (black line, n =37) and endothelial cells (blue line, n =33). C = C -value. Full size image We next explored eGFP–anillin expression in cardiomyocytes in the BZ and in intact myocardium at d4 and d12 post cryoinjury or LAD, and found only very few positive cells (0–5 cardiomyocytes per mm BZ ( Fig. 8d , arrow). Most importantly, when analysing the BZ of cryoinfarcted hearts at the two different time points ( n =7), we could not detect a single cardiomyocyte with an eGFP–anillin + midbody or contractile ring (a total of ca. 360,000 BZ cardiomyocytes was counted, ranging from 28,000 to 70,000 cardiomyocytes per heart). In clear contrast, numerous (249) BZ cardiomyocytes with nuclear eGFP–anillin expression could be identified; the number of eGFP–anillin + BZ cardiomyocytes increased from d4 to d12 post injury (0.4233±0.2153 to 1.860±0.4904 cardiomyocytes per mm BZ). These data suggest that cardiomyocytes in the adult heart do not divide in response to injury. Rather, nuclear eGFP–anillin expression in BZ cardiomyocytes indicated that these cells re-enter the cell cycle without progressing to cytokinesis. Co-staining with anti-eGFP and Ki-67 antibodies confirmed that all eGFP + cardiomyocytes were also Ki-67 + ( Fig. 8e ). The nuclear localization of eGFP–anillin implied an increase of the DNA content in cardiomyocytes via endoreduplication, which has been proposed to occur in humans after myocardial infarction [18] , [19] . Our first approach to estimate ploidy was the assessment of the nuclear area of eGFP–anillin + and eGFP–anillin − cardiomyocytes yielding significantly higher values in eGFP–anillin + cardiomyocytes ( Fig. 8f ). Next, we used confocal microscopy to determine nuclear DNA content ( Supplementary Methods ). This revealed that eGFP–anillin + cardiomyocytes in the BZ of the infarct displayed a clear increase in DNA content compared with eGFP–anillin − cardiomyocytes and endothelial cells; non-cardiomyocyte cells are known to display a diploid DNA content [20] and this was in accordance with our data ( Fig. 8g,h ). Taking the 2C DNA content of endothelial cells as a reference, the majority of eGFP–anillin − cardiomyocytes were found to have a 4C DNA content, whereas eGFP–anillin + cardiomyocytes had a DNA content between 4C and 8C. This indicated that these cells are in the endo S-phase of the endocycle ( Fig. 8i ), progressing from a 4C to 8C DNA content. Thus, cardiomyocytes do not divide after injury, but re-enter the cell cycle and undergo endoreduplication. We have established a novel, fluorescence-based system, which enables direct visualization and discrimination of late M-phase, cytokinesis and cell separation in live cells at high spatiotemporal resolution. This system relies on the fusion of eGFP with anillin, a scaffolding protein of the contractile ring. A critical feature of anillin in the context of a cell cycle phase marker is its ubiquitination by the APC Cdh1 and degradation after cell division. Thus, anillin is absent in quiescent, post-mitotic cells, an important attribute of a marker of cell cycle activity and cell division. Moreover, the subcellular localization of anillin is phase-dependent in non-quiescent cells, enabling its use to distinguish between the potential outcomes of progression into S-phase, acytokinetic mitosis or endoreduplication, and cell division. Currently, there are no live cell methods that clearly distinguish between these outcomes. As a consequence, current methods result in a marked overestimate of authentic mitosis in cells that undergo cell cycle progression without cytokinesis. In cardiac biology, for example, this most likely underlies the dramatic differences reported for cardiomyocyte renewal in intact myocardium ranging from 0.45% [21] to 40% [22] in humans and from 1 (ref. 23 ) to 80% [24] in mice. We tested the function of the system in murine and human ESCs, and show that eGFP–anillin is a specific marker for M-phase and cell division in undifferentiated and differentiated cells of all germ layers. Localization of eGFP–anillin to contractile rings and midbodies enabled discrimination between cytokinesis, and endoreduplication and acytokinetic mitosis; this was directly demonstrated with the TS cell/differentiating TGC system, an established model for endoreduplication. We also used this system to quantify cell cycle duration and length of endocycles, which were in accordance with those reported in the literature [11] , [25] . In all investigated cell types, the contractile ring persisted for approximately 20–40 min and the midbody for up to 2 h, facilitating the identification of proliferating cells even after cell division. We generated transgenic mouse lines to evaluate the system in vivo and to address two important cell biological issues: the determination of post injury myogenesis in the adult heart and the location and timing of neurogenesis during development. Proliferating and dividing cells were easily detected in tissue sections based on the presence of eGFP–anillin + midbodies and contractile rings in all tissues of transgenic embryos providing a simple and specific assay without complicated staining procedures. To distinguish between cardiomyocytes and other cell types, we crossed eGFP–anillin with αMHC–mCherry mice. This enabled monitoring of cell cycle kinetics of individual embryonic cardiomyocytes in whole organ cultures at high spatiotemporal resolution, whereas this could only be assessed by indirect methods previously [26] . We found that duration of the early G1-phase is surprisingly short in embryonic cardiomyocytes and in other cardiac cells. We also reassessed the critical question regarding the potential plasticity of terminally differentiated cardiomyocytes upon myocardial injury in eGFP–anillin mice, an area of persistent controversy [16] . We observed robust proliferation of cardiac myofibroblasts following myocardial injury [27] . In contrast no cardiomyocyte ( n =7 hearts, approximately 360,000 cardiomyocytes analysed) displayed eGFP–anillin expression in midbodies or contractile rings within the BZ of the infarct. Assuming a cell cycle duration of 24 h and persistence of the eGFP–anillin signal in contractile rings/midbodies for at least 1 h, screening of less than 24 eGFP–anillin + cardiomyocytes would be required to detect a dividing cardiomyocyte and this can be ruled out by our data. In all hearts, we observed eGFP–anillin + cardiomyocytes in the BZ of the lesion with exclusive nuclear localization of the signal ( n =249). This, as well as the observed increase in nuclear size and Ki-67 + co-staining, suggested that these cells had undergone endoreduplication and become polyploidic. This is supported by our measurements of DNA content, which revealed that the eGFP–anillin + cardiomyocytes were in S-phase of the endocycle and increased their DNA content from an average of 4C to 8C. This has been also suggested for human hearts post-myocardial infarction and clearly rules out prominent plasticity of adult cardiomyocytes. Our results do not support earlier reports on high turnover rates in mouse hearts due to multiple mitotic cardiomyocytes [28] . Furthermore, our data also demonstrate the clear advantage of the eGFP–anillin system, as it enables identification and quantitation of cell division ex vivo and in vivo . Moreover, it makes the identification, isolation and characterization of endoreduplicating cardiomyocytes possible. Determination of the sequence and extent of late-stage neurogenesis in the embryonic brain is important to better understand origins and fates of neural progenitors in the VZ and SVZ [29] of the neuroepithelium. We demonstrate that the cleavage orientation in RG and BP cells can be determined by live-cell imaging in acute brain slice preparations, information relevant to the prediction of subsequent cell fate [4] , [6] . Furthermore, this approach allowed quantitation of various cell cycle phases, which could enable the identification of distinct progenitor populations [30] . As the inheritance of the apical midbody to specific RG cells can be monitored in vivo , the eGFP–anillin system is suitable to gain insight into fate choices in neural stem and progenitor cells [5] , and into asymmetric versus symmetric division. Altogether, the eGFP–anillin system precisely marks late stages of the cell cycle and clearly identifies dividing cells versus those with cell cycle variations. Besides its use for developmental biology and regenerative medicine, it provides an excellent tool for in vitro screening approaches testing small molecules and factors modulating the cell cycle. Generation of the CAG–eGFP–anillin expression cassette Mouse anillin–cDNA was isolated by RT–PCR of total RNA from murine, embryonic diaphragm (primers: (1) 5′-GCCTGCACTCACTTCTTTCC-3′, (2) 5′-GACTATGCAGGCCCAAATGT-3′). A BglII–HpaI fragment was inserted into the multiple cloning site of the pEGFP-C1 vector (CLONTECH Laboratories, Inc.). The eGFP–anillin fusion fragment was ligated into the CAG-pDsRed2-C1 vector, thereby exchanging the DsRed2 reporter. The CAG promoter originated from the pCIG2 plasmid (kindly provided by C. Schuurmans, Calgary, Canada). A linker PCR (primers: (1) 5′-GGATCCGACCCGTTTACCGAGAAGTTG-3′, (2) 5′-GCTCCCACTTCAATTTTGTCAGAACAAC-3′) was used to introduce the first 30 amino acids into the plasmid, that were not covered by the BglI–HpaI fragment, leading to the expression of full-length eGFP–anillin. Live-cell imaging of murine and human pluripotent cells Murine ESCs and human lentiviral-transduced iPSCs were plated on fibroblast-coated glass coverslips and cultivated with ESC/iPS medium. TS cells were plated on Lumox 35 dishes (Sarstedt). Live-cell imaging was performed in a chamber with 37 °C, 5% CO 2 under a fluorescent microscope (Axiovert 200M, Carl Zeiss MicroImaging, Inc.) using the Colibri system (blue and white light-emitting diodes), a GFP filter and a X40 oil-objective. Pictures and movies were generated with the Axiovision Rel. 4.8 software (Zeiss). Murine ESCs and human iPSCs were monitored for 48 h and pictures taken every 5 min; differentiating TS cells were monitored for 48 h and pictures taken every 30 min. Human lentiviral-transduced ESCs were seeded on matrigel-coated glass coverslips and cultivated with conditioned medium. Live-cell imaging was performed in a chamber with 37 °C, 5% CO 2 under a fluorescent microscope (Axio Observer Z.1, Carl Zeiss MicroImaging, Inc.) using the Exfo x-cite 120q fluorescence light source, a GFP filter and a X20 air objective. Pictures and movies were documented with a Hamamatsu OrcaER C4742-80-12AG camera and generated with the Volocity 5.2.1 software (Perkin Elmer). Measurements of cell cycle durations were done on time-lapse sequences. Two-photon live imaging of embryonic hearts Two-photon imaging was performed with a laser-scanning microscope (SP5; Leica, Mannheim, Germany) equipped with a pulsed infrared laser (MaiTai; Spectra Physics, Darmstadt, Germany). Two-photon absorption was achieved by excitation of the fluorochromes with femtosecond pulses of infrared light with repetition rates of 80 MHz [31] . Embryonic hearts (E11.5) were placed in a tempered submerge recording chamber (Luigs-Neumann, Germany) and perfused at 35 °C with carbogen-oxygenated IMDM (Invitrogen) supplemented with 0.1 mM non-essential amino acids (Invitrogen), 50 μg ml −1 each penicillin and streptomycin (Invitrogen), 0.1 mM β-mercaptoethanol (Sigma) and with 30 mM 2,3-butanedione monoxime (BDM; Sigma) to inhibit contraction. Embryonic heart tissue was mechanically fixed by a U-shaped platinum wire stringed to nylon threads. Before eGFP–anillin time-lapse imaging, we checked for co-localization of the fusion protein with the MHC (major histocompatibility complex) reporter mCherry; for this purpose, initially two separate xyz scans for mCherry and eGFP–anillin were performed. The excitation wavelength was 790 and 920 nm, and the laser power at the tissue ~100 and ~140 mW for mCherry and eGFP–anillin, respectively. Separation of red and green light emission was achieved by a dichroic mirror (560 nm) and a band pass filter for green light (525/50 nm) in front of one of the two non-descanned detectors. Subsequent eGFP–anillin live imaging was only performed at 920 nm excitation without optical filtering. Strong eGFP–anillin emission in addition to a faint mCherry signal were observed. Volumes of 258×258×135 μm (x,y,z) were scanned in 6-min intervals for up to 6:35 h. Individual x–y planes were recorded every 2 μm (z). The thickness of an optical section was below 250 nm. Confocal imaging on acute brain slices Brain slices of E14 embryos were cut in 300-μm thickness on a vibratome (Leica) after embedding in 3% low-melting agarose, collected in complete Hank's balanced salt solution and fixed with a collagen matrix (Nitta, Japan) in a 5 cm Petri dish. Imaging was performed on an upright confocal laser-scanning microscope (FV1000, Olympus) with a X25 XPLAN N water-dipping objective (numerical aperture 1.05). During imaging, slices were cultured in Neurobasal medium plus supplements (B27, N2), incubated at 37 °C and floated with 40% O 2 and 5% CO 2 . Confocal stacks were taken at different time intervals between 1 and 15 min over a duration up to 8 h. The pinhole was opened to 300 or 500 μm during imaging. Myocardial infarction Transmural myocardial infarctions were generated in 8- to 12-week-old CAG–eGFP–anillin mice, which were anaesthetized, intubated and ventilated. The heart was exposed by thoracotomy. Cryolesions at the anterolateral left ventricular wall were generated using liquid-nitrogen-cooled copper probes 3 mm in diameter [17] . For ligations, the LAD coronary artery was occluded directly distal of the left atrial auricle, the thorax was closed by consecutive suture [17] . All animal experiments were approved by the local authorities. Histology and immunofluorescence staining All cell lines were fixed with 4% paraformaldehyde (PFA) in PBS. Adult transgenic mouse hearts were perfused with 12 ml of 4% PFA at room temperature (RT) and fixated over night at 4 °C. Organs and embryos were immersion fixed in 4% PFA over night at 4 °C. All tissues were incubated in 20% sucrose in PBS before cryopreservation in Tissue Tek O.C.T. compound (Sakura Finetek Europe B.V.). Cryopreserved embryos or adult tissues were sectioned with a cryotome CM 3050S (Leica) into 10–20 μm thick slices. Fixated cells and tissue slices were stained with the following antibodies (for 2 h at RT in 0.2% Triton X in PBS, 5% donkey serum): α-actinin (1:400, Sigma-Aldrich), Troma-1 (1:50, R. Kemler, Freiburg), TuJ1 (1:1,000, Covance), Asmac (1:800, Sigma-Aldrich), eGFP, Living Colors (1:100, Clontech), anti-GFP (1:1,000, Sigma), Tbr2 (1:200, Chemicon), BLBP (1:100, Millipore), pHH3 (1:100, Upstate Biotech), Ki-67 (1:400, kindly provided by J. Gerdes, Kiel), Ki-67 MIB-1 (1:200, Covance), phospho-vimentin (IgG1, 1:100, MBL) and Aurora-B kinase (1:400, Abcam). Primary antibodies were visualized by secondary antibodies conjugated to Cy2, Cy3 and Cy5 (1:400, Jackson ImmunoResearch) diluted in 1 μg ml −1 Hoechst 33,342 in PBS at RT for 1 h. Staining for Ki-67 in tissue slices was preceded by antigen retrieval in 10 mM sodium citrate buffer, pH 7.4. Pictures were taken with an inverted fluorescence microscope (Axiovert 200, Carl Zeiss MicroImaging, Inc.) using filters for DAPI, GFP, Cy3 and Cy5, X25, X40 and X63 DIC Plan Apochromat oil objectives, an ebx 75 light source and an AxioCam MRm digital camera. Pictures were generated with the Axiovision Rel. 4.8 software (Zeiss). Flow cytometry For flow cytometry analysis, undifferentiated mESCs were cultivated on gelatine-coated tissue culture dishes with mESC medium for at least three passages to dispose fibroblasts, washed with PBS and then dissociated to a single-cell suspension by trypsin treatment for 3–5 min. The reaction was stopped with ESC medium. After centrifugation (210 g , 5 min), the cells were washed in PBS and fixated (2% PFA at RT for 30 min or in 70% ethanol at −20 °C for 1 h). Differentiated EBs (d3–d9) were dissociated as described above and fixated with PFA or 70% ethanol. For all flow cytometric measurements, a Canto II cytometer (Becton-Dickinson) was used. Flow cytometric quantitation of eGFP–anillin + /Ki-67 + cell populations was performed by analysis of n =2 differentiation experiments using FlowJo (TreeStar). Gates were set according to isotype controls for Ki-67 stainings and autofluorescence of non-transgenic G4 ESC for eGFP–anillin fluorescence. Quantification and statistical analysis The percentual distribution of eGFP–anillin localization in CAG–eGFP–anillin ESC colonies was determined by counting at least 200 cells from three different colonies. Quantitation of eGFP–anillin-positive, Ki-67-positive, pHH3-positive and double positive cells from undifferentiated ESCs was performed on cells from n =3 CAG–eGFP–anillin clones. For the quantitation of differentiated cells from CAG–eGFP–anillin ESC clones, n =3 experiments were performed for d12 and n =1 experiment was performed for d16. A minimum of 500 cells was counted per experiment. In cryosections of infarcted CAG–eGFP–anillin hearts, the intact area of myocardium was distinguished from the infarcted area by autofluorescence using a FITC/TRITC filter. The BZ was determined as the area including all cells within a distance of 500 μm from the infarct area. Cardiomyocytes were either identified by cross-striation in the DIC image or α-actinin staining. eGFP–anillin + cardiomyocytes were identified based on clearly detectable fluorescence signals using a GFP filter set. Cardiomyocytes in the BZ of cryo- and LAD-infarcted animals were counted as follows: LAD d4 n =3 mice, 8,521 cardiomyocytes; LAD d12 n =3 mice, 9,852 cardiomyocytes. Hearts with cryolesion (CI) were used for quantitation of eGFP–anillin + cardiomyocytes, because of the reproducible lesion size and clear demarcation of the BZ: CI d4 n =3 mice, 154,236 cardiomyocytes (ranging from 37,000 to 72,000 per heart); CI d12 n =4 mice, 208,607 cardiomyocytes (ranging from 28,000 to 72,000 per heart). In Hoechst-stained sections of CI and LAD, d4 and d12 hearts nuclear areas were measured either inside (eGFP–anillin + cardiomyocytes; n =63) or outside (eGFP–anillin − cardiomyocytes; n =117) the BZ. To test for statistical significance a two-tailed, unpaired t -test with a confidence interval of 95% was used. P -values <0.05 were considered statistically significant. How to cite this article: Hesse, M. et al . Direct visualization of cell division using high-resolution imaging of M-phase of the cell cycle. Nat. Commun. 3:1076 doi: 10.1038/ncomms2089 (2012).